The key role of vibrational entropy in the phase transitions of dithiazolyl-based bistable magnetic materials The neutral radical 1,3,5-trithia-2,4,6-triazapentalenyl (TTTA) is a prototype of molecule-based bistable materials. TTTA crystals undergo a first-order phase transition between their low-temperature diamagnetic and high-temperature paramagnetic phases, with a large hysteresis loop that encompasses room temperature. Here, based on ab initio molecular dynamics simulations and new X-ray measurements, we uncover that the regular stacking motif of the high-temperature polymorph is the result of a fast intra-stack pair-exchange dynamics, whereby TTTA radicals continually exchange the adjacent TTTA neighbour (upper or lower) with which they form an eclipsed dimer. Such unique dynamics, observed in the paramagnetic phase within the whole hysteresis loop, is the origin of a significant vibrational entropic gain in the low-temperature to high-temperature transition and thereby it plays a key role in driving the phase transition. This finding provides a new key concept that needs to be explored for the rational design of novel molecule-based bistable magnetic materials. Recent years have witnessed a growing interest in the use of organic radicals as building blocks for functional molecular materials [1] , [2] , [3] , [4] , [5] . In this context, bistable materials (that is, materials that exist in two interchangeable phases under identical conditions) are being intensively pursued for their potential applications as thermal sensors as well as memory and switching devices [6] . Most of the bistable compounds so far reported are based on transition metal ions [7] , [8] , [9] , but recent work [10] strongly suggests that organic radicals can also be at the forefront in the design and fabrication of the next generation of sensors and devices. Indeed, thiazyl- [11] , [12] , spiro-biphenalenyl- [13] and nitroxide-based radicals [14] , [15] have furnished striking examples of metal-free bistable materials whose phase transitions are accompanied by changes in the magnetic, optical and/or electrical response. Several π-stacked 1,3,2-dithiazolyl (DTA) radicals have been shown to feature spin-transition behaviour between a low-temperature (LT) diamagnetic slipped stack of π-radical pairs and a high-temperature (HT) paramagnetic regular π-stack [16] . Some of these magnetic phase transitions are associated with a hysteretic behaviour [11] , [12] , [16] , [17] , [18] , [19] (thus giving rise to a region of bistability), while other transitions occur without hysteresis [20] , [21] . In addition to these intriguing solid state phase transitions, many other members of the key family of thiazyl radicals show remarkable conductivity and magnetic properties [16] , [22] , [23] , [24] , [25] . Although the properties of bistable thiazyl-based materials are reminiscent of the properties exhibited by Fe(II) spin-crossover complexes [7] , [26] , the first type of materials are not so well understood. Despite the substantial efforts recently devoted to thiazyl-based spin-transition materials, there are several crucial aspects concerning their solid state structure and the mechanisms of the phase transitions that remain largely unsettled. Two of these crucial issues are the factors that control the suppression of the spin-Peierls instability in the paramagnetic HT phases of DTA-based crystals, and the nature of the driving force of the corresponding phase transitions. Herein, we address and resolve these two pressing issues. In doing so, not only do we show that they are in fact two faces of the same coin but also we uncover that the hitherto ignored thermal fluctuations and unique dynamics of the paramagnetic phase of switchable DTAs constitute a new key element to be reckoned with when rationalizing the fascinating physico-chemical properties of DTA-based materials. The neutral radical 1,3,5-trithia-2,4,6-triazapentalenyl [27] (TTTA, Fig. 1a ) is one of the most studied molecules among the family of DTA radicals. The TTTA radical is a doublet, whose unpaired electron is formally ascribed to the deprotonated N atom in the five-membered dithiazolyl ring (inset in Fig. 1a ). However, EPR studies on dilute solutions indicate that the unpaired electron is partly delocalized over both heterocyclic rings [27] , [28] . The crystal of TTTA undergoes a first-order phase transition that results in a drastic change in the magnetic and optical response of the compound [11] , [28] , [29] . This transition occurs with a thermal hysteresis loop over a temperature interval ranging from ∼ 230 K to ∼ 310 K ( Fig. 1a ). This means that TTTA is a bistable material within an exceptionally large temperature range that encompasses room temperature. Furthermore, the phase transition of TTTA can also be driven by light irradiation [30] , [31] , [32] , [33] and the application of pressure [34] . For all these reasons, TTTA has become a prototypical molecule-based bistable material. 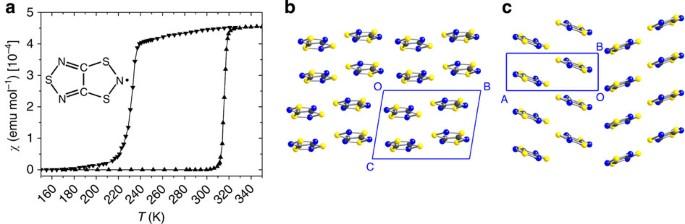Figure 1: Room-temperature magnetic bistability of TTTA-based organic material. (a) Temperature dependence of the paramagnetic susceptibility for the TTTA material on cooling (downward triangles) and on heating (upward triangles). The inset shows the molecular structure of a TTTA neutral radical; (b) Crystal packing of the triclinic LT phase of TTTA (CCDC refcode=SAXPOW06) at room temperature, viewed alonga; (c) Crystal packing of the monoclinic HT phase of TTTA (CCDC refcode=SAXPOW05) at room temperature, viewed alongc. Figure 1: Room-temperature magnetic bistability of TTTA-based organic material. ( a ) Temperature dependence of the paramagnetic susceptibility for the TTTA material on cooling (downward triangles) and on heating (upward triangles). The inset shows the molecular structure of a TTTA neutral radical; ( b ) Crystal packing of the triclinic LT phase of TTTA (CCDC refcode=SAXPOW06) at room temperature, viewed along a ; ( c ) Crystal packing of the monoclinic HT phase of TTTA (CCDC refcode=SAXPOW05) at room temperature, viewed along c . Full size image On heating above the bistability temperature range of TTTA, only the HT paramagnetic phase is observed. On cooling below the bistability range, in turn, the LT diamagnetic phase is exclusively detected. The two polymorphs of TTTA belong to different space groups (the HT phase is monoclinic, while the LT phase is triclinic) and their crystal packings feature notable differences ( Fig. 1b,c , Supplementary Note 1 and Supplementary Figs 1–4 ) [11] , [28] , [29] . The columns of radicals present in the LT phase are distorted π-stacks that comprise slipped pairs of nearly eclipsed radicals. By contrast, the columns of the HT phase are regular π-stacks of radicals, where each molecule exhibits a slipped overlap with its two adjacent molecules along the stacking direction. Besides, the TTTA molecules of the LT polymorph are all arranged in parallel planes, whereas the HT polymorph includes two distinct molecular-plane orientations. Despite numerous experimental (and also computational) studies on the TTTA material [11] , [27] , [28] , [29] , [30] , [31] , [32] , [33] , [34] , [35] , [36] , [37] , [38] , [39] , it is not yet known what prevents the radicals of the regular stacks of HT from dimerization. In addition, the nature of the driving force for the LT→HT phase transition has not yet been deciphered. Here, on the basis of extensive ab initio molecular dynamics (AIMD) simulations [40] , [41] , in conjunction with X-ray diffuse scattering measurements, we uncover that the regular stacks observed in the HT phase are in fact the average structures of a system presenting large thermal fluctuations by virtue of a fast pair-exchange dynamics occurring within the columns. This mechanism is akin to the A–H···B↔A···H–B hydrogen-bond dynamics featured by some hydrogen-bonded systems. We also demonstrate that this unique dynamics is a major source of vibrational entropy and plays a prime role in driving the LT→HT phase transition. This mechanism is very likely to be operative in other DTA-based bistable or switchable materials [17] , [18] , [19] , [20] , [21] . Model systems An appropriate model to scrutinize computationally the structure and dynamics of the LT polymorph is the triclinic supercell shown in Supplementary Fig. 5 , while for the HT polymorph is the monoclinic supercell of Supplementary Fig. 6 . Both supercells comprise eight stacks of radicals, each of them containing four radicals. The two supercells hence comprise a total of 32 TTTA molecules. These supercells allow for a balanced description of both phases and are large enough to accommodate the important thermal fluctuations of the crystal. Periodic boundary conditions in all three directions have been imposed in the simulations. Optimum structure of the LT and HT polymorphs at 0 K We first performed variable-cell geometry optimizations at 0 K for both phases of TTTA. The optimized geometries of the LT and HT phases are hereafter referred to as LT-0 and HT-0, respectively. The optimized LT-0 polymorph is nearly identical to the X-ray resolved structure at 300 K (LT-300), which is characterized by the presence of dimers within the stacks ( Fig. 2 , Supplementary Table 1 , Supplementary Fig. 7 and Supplementary Note 2 ). The slightly shorter distances between radicals in LT-0 as compared with the experimental LT-300 structure are obviously due to the thermal expansion of the crystal at finite temperatures. 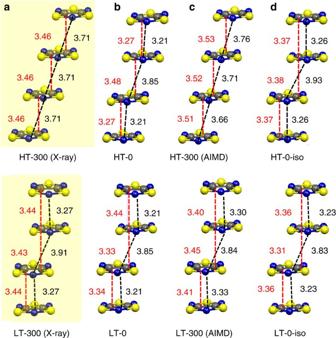Figure 2: Lateral view of one stack in both polymorphs of TTTA. The figure displays (a) the X-ray structure at 300 K, (b) the optimized structure at 0 K, (c) the average structure as obtained from the AIMD simulations done at 300 K and (d) the optimized structure of one isolated stack. The top and bottom panels correspond to the HT and LT phases, respectively. Note that the HT-0-iso and LT-0-iso have been obtained from static calculations of an isolated stack using the same supercell parameters as the ones employed in the calculation for HT-0 and LT-0. This particular set-up thus imposes the same periodic boundary conditions along the stacking direction as the ones imposed for the HT-0 and LT-0 calculations, while keeping the studied column isolated from its neighbouring columns. In all the depicted structures, the distances between the nitrogen atoms of the S-N-S moieties of adjacent radicals are marked in black, while the interplanar distances between adjacent radicals are marked in red. Figure 2: Lateral view of one stack in both polymorphs of TTTA. The figure displays ( a ) the X-ray structure at 300 K, ( b ) the optimized structure at 0 K, ( c ) the average structure as obtained from the AIMD simulations done at 300 K and ( d ) the optimized structure of one isolated stack. The top and bottom panels correspond to the HT and LT phases, respectively. Note that the HT-0-iso and LT-0-iso have been obtained from static calculations of an isolated stack using the same supercell parameters as the ones employed in the calculation for HT-0 and LT-0. This particular set-up thus imposes the same periodic boundary conditions along the stacking direction as the ones imposed for the HT-0 and LT-0 calculations, while keeping the studied column isolated from its neighbouring columns. In all the depicted structures, the distances between the nitrogen atoms of the S-N-S moieties of adjacent radicals are marked in black, while the interplanar distances between adjacent radicals are marked in red. Full size image In stark contrast to LT, the geometry optimization of HT leads to a HT-0 structure that is different from the X-ray resolved one at 300 K (HT-300). In particular, the stacks of the optimized HT-0 structure include slipped radical pairs with alternate short and long distances between the centroids of adjacent radicals ( Fig. 2 , Supplementary Note 3 and Supplementary Figs 7 and 8 ). Clearly, this distorted π-stack is at odds with the HT-300 experimental structure, where the separation between adjacent radicals of the same stack is always uniform. Despite the dimerization process upon geometry optimization, the final structure of HT-0 preserves not only the two distinct molecular-plane orientations of the resolved HT-300 structure but also its monoclinic symmetry ( Fig. 1 , Supplementary Table 1 , Supplementary Fig. 7 and Supplementary Note 3 ); hence, HT-0 is different from the LT polymorph. HT-0 should in fact be recognized as the LT crystal structure of the HT polymorph, not yet detected experimentally. The computed cohesive energy per TTTA molecule for the LT-0 and HT-0 phases is 18.3 and 17.6 kcal mol −1 , respectively. Therefore, at low temperatures LT-0 is the thermodynamically stable polymorph, and HT-0 could be only obtained under kinetic control. This is in line with the experimental observation that the LT→HT transition is endothermic [29] . Besides, the difference in cohesive energies between LT-0 and HT-0 is in good agreement with the transition enthalpy of ∼ 0.6 kcal mol −1 measured in DSC experiments [29] . The geometry of an isolated stack (namely LT-0-iso; Fig. 2 ) is virtually the same as the geometry of a single stack in the LT-0 crystal. Hence, the interactions between neighbouring columns in LT do not cause any appreciable structural distortion on the stacks with respect to the minimum energy geometry of an isolated stack. On the contrary, the stacks of HT-0 are slightly distorted as compared with the structure of an isolated HT-0-iso stack ( Fig. 2 ). In addition to significant differences in the interplanar distances between adjacent radicals, the TTTA radicals in the π dimers of the isolated HT-0-iso stack are completely eclipsed, whereas the radicals forming the π dimers in HT-0 exhibit a slipped overlap. It is thus clear that the interactions between neighbouring columns in HT prevent these stacks from adopting the minimum-energy structure of an isolated stack. All-electron DFT calculations on periodic systems and high-level correlated wavefunction-based (CASPT2) calculations carried out on an isolated stack of four TTTA radicals validate the previous results ( Supplementary Notes 4 and 5 , Supplementary Table 2 and Supplementary Figs 9–18 ). The CASPT2 calculations prove that the driving force for the dimerization process taking place during the optimization of HT-0 and HT-0-iso is the formation of long multicenter bonds [42] , [43] , [44] , [45] between TTTA radicals ( Supplementary Note 6 and Supplementary Fig. 19 ). Therefore, the striking conclusion that can be drawn from the static calculations at 0 K is that the structure of HT-300, which is based on a regular stack motif, does not correspond to a minimum in the PES of the system. This evidently raises a critical question: how can a structure that is not a minimum be observed in the X-ray measurements of HT at 300 K? Dynamics of the LT and HT polymorphs at 300 K The answer to this enigma is to be found in the thermal fluctuations of the system at finite temperatures. Indeed, AIMD simulations performed on the HT phase at 300 K (HT-300) disclose the presence of large-amplitude motions of the radicals up and down the stacks ( Fig. 3 ). Along these motions, radical−radical pairs are continually formed and broken on the picosecond timescale. Thus, a pair-exchange dynamics takes place, whereby a given TTTA radical is vividly exchanging the adjacent TTTA neighbour (upper or lower) with which it forms the eclipsed TTTA dimer. Such dynamics is reminiscent of the A–H···B↔A···H–B hydrogen-bond dynamics observed in certain hydrogen-bonded systems, where a given bridging proton jumps rapidly between two positions [46] , [47] . However appealing a comparison between our case and hydrogen-bond dynamics is, attention should be paid to the fact that quantum effects do not probably play any role in the TTTA case. Remarkably, the average structure of HT-300 obtained from this AIMD trajectory is almost identical to the X-ray crystal structure ( Fig. 2 , Supplementary Fig. 20 and Supplementary Note 7 ). This proves that the regular stack obtained from X-ray for HT-300 crystal is the average structure of a crystal presenting large thermal fluctuations along the stacks. 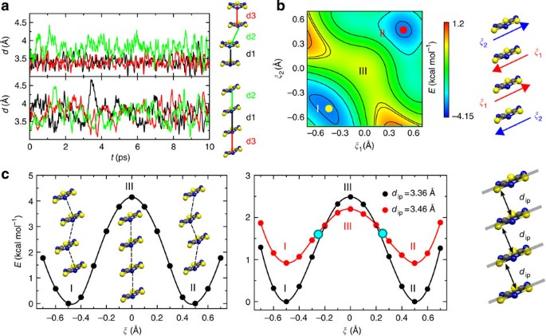Figure 3: A double-well model to rationalize the dynamics of the TTTA phases. (a) Time-resolved evolution of the distance between centroids of adjacent TTTA radicals in one of the columns of LT-300 (top) and HT-300 (bottom). (b) Potential energy surface (PES) for an isolated stack of TTTA radicals in the subspace spanned by the two geometrical variables displayed in the right-most scheme (ξ1andξ2). The sliding motion described by these variables preserves the interplanar distance between adjacent radicals (dip) within the stack. The PES has been computed with periodic boundary conditions along the stacking direction and with adipvalue of 3.27 Å (that is, the interplanar distance between adjacent radicals in HT-0). (c) Left: potential energy profile along the diagonal path connecting configurations I and II via III in the PES shown in (b), wheredip=3.27 Å. The I–III–II pathway satisfiesξ1=ξ2=ξ. Middle: potential energy profiles alongξfordip=3.36 and 3.46 Å, which correspond to the interplanar distances of LT-0 and HT-300 (or LT-300), respectively. Blue mark designates |ξ|=0.25. Note that all energy values given inb,chave been obtained with DFT calculations. Figure 3: A double-well model to rationalize the dynamics of the TTTA phases. ( a ) Time-resolved evolution of the distance between centroids of adjacent TTTA radicals in one of the columns of LT-300 (top) and HT-300 (bottom). ( b ) Potential energy surface (PES) for an isolated stack of TTTA radicals in the subspace spanned by the two geometrical variables displayed in the right-most scheme ( ξ 1 and ξ 2 ). The sliding motion described by these variables preserves the interplanar distance between adjacent radicals ( d ip ) within the stack. The PES has been computed with periodic boundary conditions along the stacking direction and with a d ip value of 3.27 Å (that is, the interplanar distance between adjacent radicals in HT-0). ( c ) Left: potential energy profile along the diagonal path connecting configurations I and II via III in the PES shown in ( b ), where d ip =3.27 Å. The I–III–II pathway satisfies ξ 1 = ξ 2 = ξ . Middle: potential energy profiles along ξ for d ip =3.36 and 3.46 Å, which correspond to the interplanar distances of LT-0 and HT-300 (or LT-300), respectively. Blue mark designates | ξ |=0.25. Note that all energy values given in b , c have been obtained with DFT calculations. Full size image As for the LT polymorph, the AIMD trajectory acquired at 300 K (LT-300) does not show such large-amplitude motions of the radicals. Consequently, in LT-300 the radical–radical pairs are preserved over simulation time ( Fig. 3 ). As in the HT-300 crystal, the average structure for LT-300 obtained from the simulations is virtually identical to the X-ray crystal structure ( Fig. 2 , Supplementary Fig. 20 and Supplementary Note 7 ). Overall, the results obtained for HT-0 can be reconciled with the X-ray-resolved HT-300 structure when taking into consideration the thermal fluctuations of the system. Which is then the origin of such pronounced fluctuations? Unveiling a 2nd-order phase transition in the HT polymorph A most valuable insight into the origin of these fluctuations is provided by the two-dimensional (2D) probability distribution functions (PDFs) associated with the d ip interplanar distance and the d sl relative slippage between adjacent radicals ( Fig. 4 ). The 2D-PDF of HT-300 presents a single broad peak with a maximum at an interplanar distance between adjacent radicals of ∼ 3.4 Å. This means that the regular spaced stack is not only the average structure but also the most probable arrangement. On the contrary, the 2D-PDF of LT-300 features two peaks: the peak with the maximum at a zero value of the degree of relative slippage corresponds to the eclipsed dimers, whereas the other peak corresponds to a slipped TTTA pair. 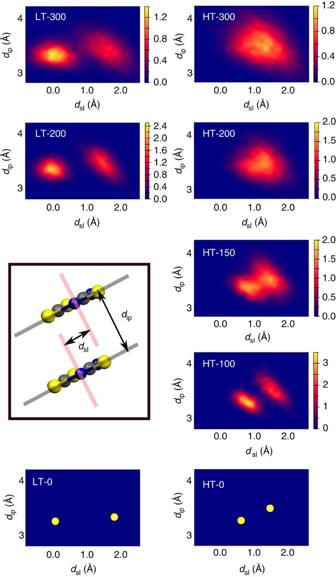Figure 4: Temperature dependence of the dynamics of the two TTTA phases. The figure displays the temperature dependence of the 2D-PDFs for the HT and LT polymorphs of TTTA in the subspace spanned by the two dominant geometrical components of the vector connecting the centroids of adjacent radicals (see inset fordipanddsl;dipmeasures the interplanar distance between adjacent radicals in one stack;dslmeasures the degree of relative slippage between adjacent radicals of the stack). Note that the left-most peak in the bimodal distributions corresponds to the eclipsed TTTA dimer (0<dsl<0.75). The PDFs have been obtained from the configurations sampled during the AIMD simulations. Figure 4: Temperature dependence of the dynamics of the two TTTA phases. The figure displays the temperature dependence of the 2D-PDFs for the HT and LT polymorphs of TTTA in the subspace spanned by the two dominant geometrical components of the vector connecting the centroids of adjacent radicals (see inset for d ip and d sl ; d ip measures the interplanar distance between adjacent radicals in one stack; d sl measures the degree of relative slippage between adjacent radicals of the stack). Note that the left-most peak in the bimodal distributions corresponds to the eclipsed TTTA dimer (0< d sl <0.75). The PDFs have been obtained from the configurations sampled during the AIMD simulations. Full size image The evolution of the 2D-PDFs of LT and HT upon cooling is markedly different too ( Fig. 4 , Supplementary Fig. 21 and Supplementary Note 8 ). While the bimodal character of the PDF for LT is preserved at lower temperatures, the unimodal PDF for HT at 300 K gradually transforms into a bimodal PDF as the temperature is lowered. This reflects a change in the dynamics of the crystal. At 300 K, each TTTA within a stack is crystallographically equivalent by virtue of the fast pair-exchange dynamics described above. Such exchange dynamics at 300 K gradually slows down and ultimately freezes at 100 K. The temperature dependence of the PDFs for HT is thus a fingerprint for a second-order or order–disorder transition within the stacks upon heating ( Supplementary Note 9 ). A double-well model for the fast pair-exchange dynamics The order–disorder transition of HT and, hence, the unique dynamics featured by HT-300 can be rationalized on the basis of a double-well model potential. Let us consider an isolated stack of four TTTA radicals with periodic boundary conditions along the stacking direction. Given a regular arrangement of the radicals in the stack (configuration III in Fig. 3c ), two distinct distorted stacks are conceivable if one considers a dimerization process along the stacking direction (configurations I and II in Fig. 3c ). These three configurations can be smoothly transformed into each other by changing the geometrical variables ξ 1 and ξ 2 ( Fig. 3b ), which drive a relative sliding motion between TTTA radicals along the stack. The PES in the subspace spanned by these two variables reveals that configurations I and II are minima, while configuration III is a transition state ( Fig. 3b ). The potential energy profile ( Fig. 3c ) along the diagonal of this PES exhibits the characteristic shape of a double-well model potential, in which the maximum is associated with the regular structure observed at HT-300. At this point, it is crucial to bear in mind that the pair-exchange process described above is equivalent to converting configuration I into II (and vice versa ) via configuration III along the coordinate ξ ( Fig. 3 ). In addition, the barrier for this process strongly depends on the interplanar distance between adjacent radicals, d ip ( Fig. 3c ). Since smaller d ip values are achieved at lower temperatures, it is concluded that the barrier will decrease as the temperature increases. In fact, Fig. 3c clearly shows that the barrier for the d ip value associated with the HT-0 structure is ∼ 4 kcal mol −1 , whereas the barrier for the d ip value associated with the HT-300 structure is ∼ 1 kcal mol −1 . Concerning the HT phase, at low temperatures ( T <175 K), the thermal energy of the stacks is not large enough as to overcome the barrier separating I and II, and no jumps between minima are observed. This gives rise to the bimodal PDFs of Fig. 4 . The reverse situation is encountered upon heating up to room temperature. The thermal energy is then sufficient to convert I into II ( k B T is ∼ 0.6 kcal mol −1 at 300 K), thus yielding a unimodal distribution that is centred on the maximum of the double-well potential ( Fig. 4 ). From a physical point of view, this means that for temperatures higher than ∼ 200 K each TTTA radical stands most likely at the midpoint of the line segment connecting its two adjacent neighbours within the stack (in agreement with the regular intra-stack arrangement in HT) while undergoing important fluctuations around that point. The double-well framework applies to the LT phase too. The fact that the bimodal character of the corresponding PDFs ( Fig. 4 ) prevails up to 300 K entails that the energy barrier is substantially higher than the thermal energy (at least) up to room temperature. This of course raises a major question: why is the energy barrier in LT larger than in HT? A qualitative answer to this question is to be found in the different structures adopted by the TTTA stacks in LT-0 and HT-0. As described above, LT-0 comprises completely eclipsed dimers, whereas HT-0 contains slipped dimers. This difference is clearly reflected by looking at the distance between the two peaks in the lowest panels of Fig. 4 : the distance between the two peaks is significantly shorter in HT-0. Since the interconversion of configurations I and II is equivalent to finding a pathway between the two peaks of these graphics, it follows that such interconversion involves a shorter pathway in HT-0 than in LT-0. This means that in the profiles of Fig. 3c , the actual starting geometry in the HT pathway is not the equilibrium geometry but a point located midway between the minima (I or II) and the maximum (III) with | ξ | estimated to be ∼ 0.25 (blue mark in Fig. 3c ). This implies that the effective barrier for HT can be easily overcome (based on the red profile of Fig. 3c , our estimate is that the effective barrier for HT-300 is ∼ 0.5 kcal mol −1 ), in sharp contrast with LT-300 (whose initial geometry is the actual minima of the energy profile, at | ξ |≈0.5). Role of vibrational entropy in the LT→HT phase transition The fast pair-exchange dynamics taking place within the HT stacks is not observed in LT. This hints at a large vibrational entropy increment (Δ S vib = S vib,HT − S vib,LT ) upon the LT→HT phase transition. Exhaustive AIMD simulations prove that this is indeed the case. In these simulations, the value of T Δ S vib at any temperature can be obtained as Δ U vib −Δ A vib , where U stands for internal energy and A for Helmholtz free energy. Note that we use Helmholtz free energies because the simulations for both polymorphs have been carried out in the canonical (or NVT) ensemble. Δ U vib is directly extracted from the AIMD simulations, while Δ A vib is computed by a thermodynamic integration-based technique using the temperature dependence of Δ U vib as input data ( Supplementary Note 10 ). This methodology transcends the commonly used vibrational harmonic approximation, because it allows to capture the anharmonic effects heralded by the pair-exchange dynamics. The total variation of the entropy (Δ S tot ) and the total Helmholtz free energy variation (Δ A tot ) are obtained by adding the electronic contribution (Δ S el and Δ A el ) to Δ S vib and Δ A vib . The electronic contributions originate in the fact that LT is magnetically silent, whereas HT exhibits quenched paramagnetism ( Supplementary Note 10 ). The temperature dependence of Δ U vib , Δ A vib , Δ S vib , Δ A tot and Δ S tot for the LT→HT phase transition is displayed in Fig. 5 . The computed value of Δ U vib (0.94 kcal mol −1 ) at 310 K agrees reasonably well with the experimental transition enthalpy associated with the LT→HT transition at that temperature [29] (0.56 kcal mol −1 ). The fact that Δ U vib changes with temperature is an evidence of the relevance of the anharmonic effects ( Supplementary Fig. 22 ). Δ A tot decreases with temperature and becomes zero at ∼ 370 K, implying that the LT→HT phase transition is in equilibrium (in reasonable agreement with DSC experiments [29] , which indicate that equilibrium is within the 234–315 K temperature range). As observed in the lower panels of Fig. 5 , the temperature dependence of Δ A tot is mainly controlled by the T Δ S tot term. The computed T Δ S tot value (0.87 kcal mol −1 ) at 310 K is similar to the experimental entropic term for the LT→HT transition (0.56 kcal mol −1 ) at that temperature [29] . Note that the experimental entropic term is given under the assumption that the LT→HT phase transition at 310 K takes place in equilibrium (that is, with Δ G =0). Finally, comparison between T Δ S tot and T Δ S vib shows that the vibrational entropy (stemming from the fast intra-stack dimer exchange in HT) is a key contribution to the total entropy increase in going from LT to HT. Therefore, our results bring to light that vibrational entropy is crucial to enable the LT→HT phase transition. 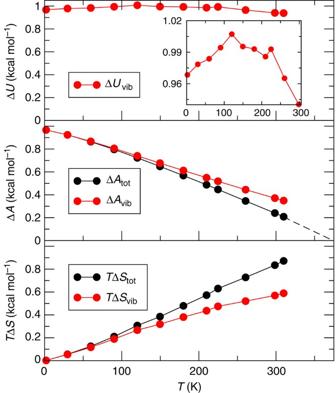Figure 5: The importance of vibrational entropy in the phase transition of TTTA. Temperature dependence of the difference in internal energy (ΔU, top), Helmholtz free energy (ΔA, middle) and entropy (ΔS, bottom) between the HT and LT phases of TTTA. If we denote any of the thermodynamic magnitudes herein considered byX, ΔXis defined asXHT−XLT. ΔXvibrefers to the vibrational contribution of ΔX, while ΔXtotrefers to the sum of the vibrational and electronic contributions. The solid lines connect the points to guide the eye. The inset in the upper panel is a magnification of the ΔUcurve. The dashed line in ΔAis an extrapolation of the parabola that best fits the ΔAvalues, employed here to estimate the temperature at which ΔAtot=0. Figure 5: The importance of vibrational entropy in the phase transition of TTTA. Temperature dependence of the difference in internal energy (Δ U , top), Helmholtz free energy (Δ A , middle) and entropy (Δ S , bottom) between the HT and LT phases of TTTA. If we denote any of the thermodynamic magnitudes herein considered by X , Δ X is defined as X HT − X LT . Δ X vib refers to the vibrational contribution of Δ X , while Δ X tot refers to the sum of the vibrational and electronic contributions. The solid lines connect the points to guide the eye. The inset in the upper panel is a magnification of the Δ U curve. The dashed line in Δ A is an extrapolation of the parabola that best fits the Δ A values, employed here to estimate the temperature at which Δ A tot =0. Full size image Experimental confirmation of thermal fluctuations In order to confirm the validity of the previous theoretical results, X-ray experimental studies were performed for HT and LT polymorphs searching for the presence of diffuse structure in the X-ray diffraction patterns. The significant diffuse scattering detected in the single-crystal X-ray diffraction ω oscillation photographs of the HT phase at 300 K ( Fig. 6 and Supplementary Fig. 23 ), together with the temperature dependence of the diffuse structure of the Bragg spots ( Supplementary Figs 24 and 25 ), support the large thermal fluctuations observed in the simulations. Moreover, the excellent agreement between the computed average structures and the X-ray crystal structure for both HT-300 and LT-300, in conjunction with the good agreement between the computed and experimental thermal ellipsoids of the atoms of the TTTA molecules in both polymorphs (specially for HT-300; Fig. 6 , Supplementary Figs 26 and 27 , Supplementary Tables 3 and 4 and Supplementary Note 11 ) provide further evidence of the quality of the AIMD trajectories obtained. 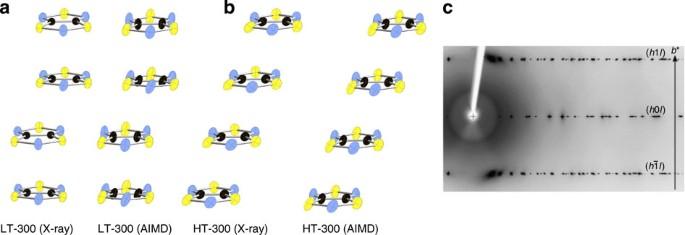Figure 6: Experimental support of the large thermal fluctuations in TTTA. Comparison between the thermal ellipsoids of the atoms of the TTTA molecules obtained from the X-ray measurements and those obtained from the AIMD simulations for both (a) LT-300 and (b) HT-300 polymorphs. The displayed ellipsoids correspond to a probability of 50%. (c) Single-crystal X-ray diffractionωoscillation photograph for HT-300 (the vertical direction is along the stacking direction). Figure 6: Experimental support of the large thermal fluctuations in TTTA. Comparison between the thermal ellipsoids of the atoms of the TTTA molecules obtained from the X-ray measurements and those obtained from the AIMD simulations for both ( a ) LT-300 and ( b ) HT-300 polymorphs. The displayed ellipsoids correspond to a probability of 50%. ( c ) Single-crystal X-ray diffraction ω oscillation photograph for HT-300 (the vertical direction is along the stacking direction). Full size image When solving the structure of the HT phase of TTTA by direct methods and standard differential map techniques, large residual electron densities around the atoms are revealed ( Fig. 7a ). Although the diffuse scattering measurements demonstrate that these residual densities arise from dynamic disorder, it is very instructive to refine the HT-300 phase assuming that they arise from static disorder. If we assume a 50:50 occupancy disorder between two extreme structures, the yellow circles of Fig. 7b would mark the atom positions in both extreme structures. These yellow circles would result in the two extreme molecular configurations displayed in Fig. 7c . It is exceedingly important to realize ( Fig. 7d,e ) that these two refined extreme structures are compatible with the two distorted stacks involved in the pair-exchange dynamics process (configurations I and II in Fig. 3c ). Since the dynamic disorder necessarily implies the presence of a dynamic conversion between the two refined extreme structures, and these extreme structures are compatible with the molecular configurations involved in the pair-exchange dynamics, it follows that these two refined extreme structures constitute another proof of the presence of this unique dynamics. 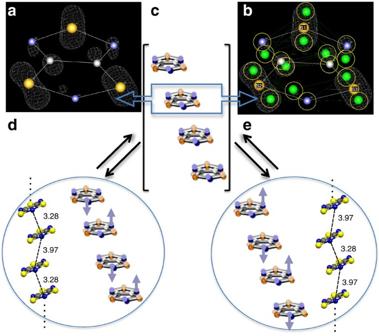Figure 7: Experimental support of the pair-exchange dynamics in TTTA. (a) Residual electron density (white mesh) around the atom positions of a TTTA radical in the HT phase. (b) Atom positions within the corresponding electron density mesh giving as a result two extreme structures, as indicated by yellow circles. (c) Extreme structures of the HT phase of TTTA determined experimentally under the assumption of static disorder (R1 (I>2.00σ(I))=0.0661;R(all)=0.0675;wR2 (all)=0.1802; GOF=1.104; occupancy factors 54:46). These two extreme structures are compatible with the distorted radical stacks found upon DFT optimization of a four-radical periodic model, shown indande. Note that these extreme structures result from an intra-stack pairing process of the experimental (c) structure, as schematically represented by arrows. Figure 7: Experimental support of the pair-exchange dynamics in TTTA. ( a ) Residual electron density (white mesh) around the atom positions of a TTTA radical in the HT phase. ( b ) Atom positions within the corresponding electron density mesh giving as a result two extreme structures, as indicated by yellow circles. ( c ) Extreme structures of the HT phase of TTTA determined experimentally under the assumption of static disorder ( R 1 ( I >2.00 σ ( I ))=0.0661; R (all)=0.0675; wR 2 (all)=0.1802; GOF=1.104; occupancy factors 54:46). These two extreme structures are compatible with the distorted radical stacks found upon DFT optimization of a four-radical periodic model, shown in d and e . Note that these extreme structures result from an intra-stack pairing process of the experimental ( c ) structure, as schematically represented by arrows. Full size image Finally, it is worth mentioning that most recent terahertz (THz) time-domain spectroscopy measurements [48] have revealed that the vibrational spectra of LT and HT are markedly different in the THz region. Elegant studies [48] have demonstrated that these differences can be exploited to monitor the phase transition of TTTA, which implies that THz spectroscopy can provide new insights into the dynamics and mechanism of this phase transition. Since the THz bands detected in these experiments correspond to intermolecular vibrations of TTTA molecules, we can conclude that the different vibrational spectra of LT and HT in the THz region is in line with our finding that the dynamics featured by the TTTA molecules in the two phases are distinct ( Fig. 3a ). Indeed, our computational analysis shows that the different dynamics give rise to significant differences in the vibrational density of states of LT and HT in the THz region (see Supplementary Note 12 and Supplementary Fig. 28 for further details). The large-scale AIMD simulations and new X-ray measurements on the TTTA material reported above will have a profound impact on the way in which the structure and properties of this bistable material will be interpreted from now on. First of all, our results uncover that the regular stack motif of the HT polymorph does not correspond to a minimum in the PES of the system, but to the free energy surface. Instead, the optimum structure of HT at 0 K presents π-stacks that comprise slipped TTTA dimers. Upon heating up to ∼ 200 K, the HT polymorph gradually undergoes a second-order phase transition within π-stacks from an ordered (or dimerized) state into a disordered state, where each radical continually changes the neighbour with which it forms an eclipsed dimer (fast pair-exchange dynamics). This unique dynamics renders all the radicals of one stack crystallographically equivalent and, thus, explains the resolved X-ray regular stacking motif of HT in the range of 225–310 K. The reason why the second-order phase transition in HT has not been yet experimentally detected below this range is twofold: (i) at temperatures below the hysteresis loop range, LT is more stable than HT, and (ii) upon cooling, the HT→LT first-order transition occurs at ∼ 230 K, whereas the second-order transition would take place gradually at ∼ 200 K. In stark contrast to HT, the LT polymorph remains in an ordered state within the 0–310 K temperature range. This indicates that the energy barrier that controls the fast pair-exchange dynamics is higher in LT, which is a consequence of its different packing structure. The previous considerations imply that the LT→HT phase transition at ∼ 310 K is in fact a LT(ordered)→HT(disordered) phase transition. In other words, besides the cleavage/formation of intermolecular bonds between stacks associated with the first-order phase transition, the LT→HT transition brings about a transformation of ordered stacks into disordered stacks. For the same reasons, the HT→LT phase transition occurring at ∼ 230 K is in fact a HT(disordered)→LT(ordered) phase transition. Previous experimental work by Awaga and co-workers [29] concluded that the electronic entropy gain was not sufficient to counterbalance the enthalpy gain in the first-order LT→HT phase transition at ∼ 310 K. Our work reveals that the missing entropy originates in the vibrational entropy associated with the fast pair-exchange dynamics featured by the disordered HT polymorph. Therefore, the vibrational entropy plays a key role as a driving force for the LT→HT phase transition, in clear parallelism to the known scenario in Fe(II)-based spin-crossover complexes. The reported findings transcend the specific system herein studied. Our work provides novel concepts that are essential for the understanding of the properties of other dithiazolyl-based bistable materials (preliminary studies on the 3-cyanobenzo-1,3,2-dithiazolyl material [20] strongly suggest that the fast pair-exchange dynamics herein presented also applies within this class of materials). At the same time, the idea that radical dimerization should be avoided at any cost in order to obtain solids presenting useful magnetic properties should be reconsidered from the point of view of the fast pair-exchange dynamics. This concept indeed offers a new tool for the rational design of novel spin-transition and bistable materials. Finally, taking an even broader perspective, our study also questions the common idea that observed polymorphic structures are minima on the PES of crystals. As we have shown, X-ray structures can correspond to an average of two minima structures that dynamically interconvert at the working temperature. The accompanying large thermal fluctuations can in turn have a major influence on the physical properties of the system at a given temperature. In this sense, our work calls into question the validity of the common interpretation of magnetic properties based on static average structures. This crucial issue, which goes beyond the dependency of the J AB magnetic exchange coupling on the temperature, will be addressed in future studies. Computational details Plane wave pseudopotential calculations were employed for both the AIMD [40] and the geometry optimizations. These calculations were carried out using the PBE exchange–correlation functional [49] , [50] within the spin unrestricted formalism, together with Vanderbilt ultrasoft pseudopotentials [51] , and Γ-point sampling of the Brillouin zone. In all the calculations, the semiempirical dispersion potential introduced by Grimme [52] was added to the conventional Kohn–Sham DFT energy in order to properly describe the van der Waals interactions between the different TTTA molecules. The parametrization employed in our work is the so-called DFT-D2 (ref. 52 ) parametrization. It is noted that a series of recent benchmark calculations have shown that the use of PBE together with the Grimme [52] correction furnishes good predictions for the structure and cohesive energies of molecular crystals [53] . The AIMD simulations were performed using the efficient Car–Parrinello propagation scheme [41] as implemented in the CPMD package [54] . In these simulations, the plane wave basis set was expanded at a kinetic energy cutoff of 25 Ry. The molecular dynamics time step was set to 4 a.u. and the fictitious mass for the orbitals was chosen to be 400 a.u. All dynamic simulations were performed in the canonical ensemble using Nosé–Hoover chain thermostats [55] in order to control the kinetic energy of the nuclei and the fictitious kinetic energy of the orbitals. For the geometry optimizations at 0 K of both LT and HT, we used a two-step procedure. We first performed a variable-cell geometry optimization with a plane wave basis set expanded at a kinetic energy cutoff of 70 Ry. These calculations, in which the atomic positions and the lattice parameters are optimized simultaneously, were carried out with the QUANTUM ESPRESSO package [56] . The initial atomic positions and lattice parameters for the optimization of LT-0 and HT-0 were taken from the X-ray resolved structures of LT-300 and HT-300 (SAXPOW06 and SAXPOW05, respectively). The initial lattice parameters of the LT and HT supercells are collected in Supplementary Table 1 . The number of plane waves was kept constant throughout the variable-cell relaxations. A constant number of plane waves implies no Pulay stress but a decreasing precision of the calculation as the volume of the supercell increases [40] . The large cutoff employed in these calculations ensures that the artefacts arising from this change of precision are negligible. After the variable-cell relaxations, the corresponding optimized atomic positions and optimized lattice parameters for both LT-0 and HT-0 polymorphs were used to define the initial geometries for a subsequent optimization at a cutoff of 35 Ry in which the lattice parameters were kept fixed. This new optimization with a smaller cutoff was performed to be able to carry out a finite-difference normal mode analysis of the final optimized structures at a reasonable computational cost. It should be mentioned that switching from a cutoff of 70 Ry to a cutoff of 35 Ry results in negligible differences in both the structures and energies of both polymorphs. Indeed, the optimized structures of LT and HT at 35 Ry are virtually identical to the LT and HT structures at 70 Ry. In fact, the forces on all atoms of the system in the starting geometries of the calculations at 35 Ry are smaller than 8 × 10 −4 a.u. In addition, the change in energy in going from the starting geometry to the final one is less than 0.02 kcal mol −1 (given per TTTA molecule) for both polymorphs. It thus follows that the computational strategy has been properly set up. The reader is referred to Supplementary Notes 4 and 5 and Supplementary Figs 9–18 for the large number of tests that has been carried out to validate the computational methodology. Experimental details The diffraction data for the single-crystal structure analysis were collected on a Rigaku AFC-10 instrument equipped with a Saturn 70 CCD detector by using graphite-monochromated Mo Kα radiation (λ=0.710690 Å) under a cold nitrogen stream. Temperature was corrected with the thermocouple. The frame data were integrated and corrected for absorption with the Rigaku/MSC Crystal Clear package [57] . The structures were solved by direct methods (SIR-97 (ref. 58 )) and standard difference map techniques, and were refined with full-matrix least-square procedures on F 2 . The non-hydrogen atoms were refined anisotropically. Hydrogen atoms were refined using the riding model. All calculations were performed using the Crystal Structure [59] crystallographic software package except for refinement, which was performed using SHELXL-97 (ref. 60 ). How to cite this article: Vela, S. et al . The key role of vibrational entropy in the phase transitions of dithiazolyl-based bistable magnetic materials. Nat. Commun. 5:4411 doi: 10.1038/ncomms5411 (2014).